Spectroscopic and computational investigation of actinium coordination chemistry Actinium-225 is a promising isotope for targeted-α therapy. Unfortunately, progress in developing chelators for medicinal applications has been hindered by a limited understanding of actinium chemistry. This knowledge gap is primarily associated with handling actinium, as it is highly radioactive and in short supply. Hence, Ac III reactivity is often inferred from the lanthanides and minor actinides (that is, Am, Cm), with limited success. Here we overcome these challenges and characterize actinium in HCl solutions using X-ray absorption spectroscopy and molecular dynamics density functional theory. The Ac–Cl and Ac − O H 2 O distances are measured to be 2.95(3) and 2.59(3) Å, respectively. The X-ray absorption spectroscopy comparisons between Ac III and Am III in HCl solutions indicate Ac III coordinates more inner-sphere Cl 1– ligands (3.2±1.1) than Am III (0.8±0.3). These results imply diverse reactivity for the +3 actinides and highlight the unexpected and unique Ac III chemical behaviour. Understanding of the chemistry of trivalent actinides has broad-potential impacts on society through diverse areas, including cancer therapy [1] , [2] , [3] , nuclear waste [4] , [5] , [6] , energy and global security [7] . However, with the exception of U III (refs 6 , 7 , 8 , 9 ), fundamental understanding of the early-to-mid-actinides in the trivalent oxidation state (An=Ac III , Np III , Pu III , Am III , Cm III , Bk III and Cf III ) remains substantially less developed than that of the main group, transition metals and lanthanides. Significant experimental challenges associated with the highly radioactive samples, limited access to material of interest, and the redox instability of some An III ions have necessitated numerous heroic efforts to advance An III chemistry [6] , [10] , [11] , [12] , [13] , [14] , [15] . The 2015 Long Range Plan for the DOE-NP Isotope Program [16] highlighted the importance of advancing Ac III chemistry in comparison with the other An III ions. In this document, 225 Ac was identified as a promising anticancer therapeutic agent. The report focused on global interest in exploiting the α-emissions from 225 Ac and its radioactive daughters to selectively destroy the malignant cells [17] , [18] . To use these α-particles therapeutically, the 225 Ac isotope must be attached to cancer-selective targeting vectors using a stable chelating agent. Unfortunately, the limited availability of 225 Ac [t ½ =10.0(1) d; National Nuclear Data Center (NNDC)], or a useful surrogate, has impeded development of actinium chelators. For instance, the use of 227 Ac, the longest-lived actinium isotope [t ½ =21.772(3) y; NNDC] provides the best possible alternative for improving ligand design. However, the worldwide inventory of 227 Ac is currently insufficient for meeting this demand. Historically, these challenges were magnified by the electronic ground state of Ac III (5 f 0 6 d 0 ), which is essentially invisible to common spectroscopies (for example, ultraviolet–visible, fluorescence, electron paramagnetic resonance and so on). Hence, applying alternative characterization methods that account for (1) high radioactivity, (2) small samples sizes (1–30 μg) and (3) closed shell electronic configurations would facilitate innovative chelation designs for delivery of 225 Ac through the biological milieu to the targeted tumour site. Recent upgrades at the Stanford Synchrotron Radiation Lightsource (SSRL), such as the new 100-element solid-state Ge detector array on beamline 11-2, have provided new opportunities to overcome the aforementioned challenges. This capability has improved sensitivity for trace-level detection in environmental samples using X-ray absorption fine-structure (XAFS) spectroscopy [19] , [20] . While this instrumentation has been used primarily in environmental sciences, here we exploit the capability to conduct the first actinium XAFS study reported to date. Using this method, 227 Ac in concentrated HCl solutions are characterized at the Ac L 3 -edge. Our interpretations of the spectra are guided by molecular dynamics density functional theory (MD-DFT) calculations [21] , [22] , [23] , [24] , [25] . To establish confidence in the spectroscopic and computational methods, the Ac III results are compared with analogous measurements on Am III . This ion is selected because—among the redox stable trivalent actinides—its ionic radius is most similar to Ac III . Overall, this approach enables the Ac–Cl and Ac − O H 2 O distances to be measured and allows the coordination chemistry of Ac III and Am III to be directly compared. The experimental and computational data show more chloride ions in the inner coordination sphere for Ac III and the results are presented in comparison with previous actinide(III) XAFS studies. This study reveals an unexpected divergence in +3 f -element reactivity. Furthermore, the research highlights the need to better characterize An III chemistry in support of developing α-emitting therapeutic agents. X-ray absorption near-edge structure spectroscopy To evaluate Ac III and Am III binding of Cl 1– versus H 2 O, three solution-phase samples were prepared: actinium chloride (Ac III in HCl; 11 M); americium chloride (Am III in HCl; 11 M); and the americium aquo ion (Am III in HO 3 SCF 3 , 0.11 M), referred to hereafter as Ac-HCl , Am-HCl and Am-Aquo . To mitigate safety concerns associated with the 227 Ac isotope, radioactive daughters (primarily 227 Th and 223 Ra) were removed before the measurements at the SSRL synchrotron, as previously described (see Methods) [26] , [27] . The samples were then returned to Los Alamos National Laboratory before a significant quantity of the daughters re-emerged ( ∼ 10 days). The Ac and Am L 3 -edge X-ray absorption near-edge structure (XANES) spectra from Ac-HCl , Am-HCl and Am-Aquo were background subtracted and normalized ( Fig. 1 ). The spectra were similar as they contained a pronounced edge-peak superimposed on an absorption threshold. From the perspective of the free ion, the edge-feature could be crudely described as originating from electric-dipole allowed transitions from the actinide 2 p -orbitals to unoccupied states that contain actinide 6 d -character, that is, for Ac III 2 p 6 …5 f 0 6 d 0 →2p 5 …5 f 0 6 d 1 (refs 28 , 29 ). 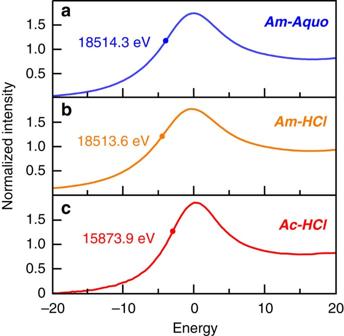Figure 1: Solution phase AcIIIand AmIIIL3-edge XANES. (a) XANES spectra forAm-Aquo(0.11 M HO3SCF3) in blue trace. (b) XANES spectra forAm-HCl(11 M HCl) in orange trace. (c) XANES spectra forAc-HCl(11 M HCl) in red trace. The actinium and americium spectra were calibratedin situto RbCl pellet (15,203.81 eV) and Zr foil (17,998 eV) respectively. Figure 1: Solution phase Ac III and Am III L 3 -edge XANES. ( a ) XANES spectra for Am-Aquo (0.11 M HO 3 SCF 3 ) in blue trace. ( b ) XANES spectra for Am-HCl (11 M HCl) in orange trace. ( c ) XANES spectra for Ac-HCl (11 M HCl) in red trace. The actinium and americium spectra were calibrated in situ to RbCl pellet (15,203.81 eV) and Zr foil (17,998 eV) respectively. Full size image The Ac L 3 -edge spectrum was of quintessential significance, as it represented the first actinium XANES measurement. The edge-peak line shape was quite broad and spanned over ∼ 30 eV, owing to the short core-hole lifetime. The peak maximum and inflection point (where first and second derivatives of the data equalled zero) were determined to be 15,877.3 and 15,873.9 eV, respectively. For the americium samples, the inflection point from Am-Aquo was found at 18,514.3 eV, which was consistent with americium in the +3 oxidation state [30] , [31] . Changing the solution matrix from HO 3 SCF 3 (0.11 M) to HCl (11 M) shifted the edge-peak inflection point to lower energy by 0.7 eV. The Am L 3 -edge energy difference was attributed to an electronic change that accompanied Cl 1– displacement of H 2 O in the Am III inner coordination sphere ( vide infra ), that is, Am-Aquo versus Am-HCl . Given the relative ease with which the Ac III and Am III L 3 -edge XANES measurements were obtained—and in light of the incompatibility of other spectroscopic techniques for probing dilute actinium samples—we anticipate that these results will provide a foundation for characterizing the coordination chemistry of actinium in other chemical environments in the future. Extended X-ray absorption fine structure Appreciable differences were observed in the solution-phase k 3 χ( k ) extended X-ray absorption fine-structure (EXAFS) data (room temperature) from solutions containing Ac-HCl , Am-HCl and Am-Aquo ( Fig. 2 ). For instance, a substantial phase shift and change in frequency in the EXAFS oscillations was observed in the spectrum from Ac-HCl in comparison with the americium spectra. The Ac-HCl spectrum was comprised of at least two substantial contributions; one characterized by a long frequency and the other by a short frequency. The presence of two frequencies was most likely associated with a significant number of both Cl 1– and H 2 O molecules in the Ac III inner coordination sphere. In contrast, for Am-HCl , the frequency of EXAFS oscillations was dominated by one major sinusoidal component, such that the Am-HCl spectrum was almost superimposable on that from Am-Aquo . The similarity between Am-HCl and Am-Aquo suggested that H 2 O molecules dominated the inner coordination sphere in Am-HCl , with Cl 1– content being slight. Overall, this comparison highlighted significant differences in Ac III versus Am III solution speciation. 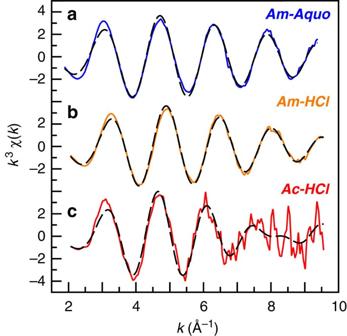Figure 2: Solution phase AcIIIand AmIIIL3-edge EXAFS. (a) EXAFSk3χ(k) spectra forAm-Aquo(0.11 M HO3SCF3) in blue trace. (b) EXAFSk3χ(k) spectra forAm-HCl(11 M HCl) in orange trace. (b) EXAFSk3χ(k) spectra forAc-HCl(11 M HCl) in red trace. Fits to the data have been provided as dashed black traces. Figure 2: Solution phase Ac III and Am III L 3 -edge EXAFS. ( a ) EXAFS k 3 χ( k ) spectra for Am-Aquo (0.11 M HO 3 SCF 3 ) in blue trace. ( b ) EXAFS k 3 χ( k ) spectra for Am-HCl (11 M HCl) in orange trace. ( b ) EXAFS k 3 χ( k ) spectra for Ac-HCl (11 M HCl) in red trace. Fits to the data have been provided as dashed black traces. Full size image The EXAFS data were fit by allowing the coordination numbers (CN), the Debye–Waller factors ( σ 2 ), and the interatomic distances ( R ) to converge to reasonable values. Limitations associated with the solution-phase room-temperature EXAFS measurements constrained meaningful data to ∼ 10 k (9, 10.5 and 12 k for solutions containing Ac-HCl , Am-HCl and Am-Aquo , respectively). As a result, scattering pathways beyond the first coordination shell (including multiple scattering pathways, for example, Cl−M−H 2 O) were not considered. To most effectively describe how the EXAFS models were obtained, it was instructive to begin with Am-Aquo , then introduce the possibility of Cl 1– ligation for Am-HCl , and conclude with the Ac-HCl . Before modelling the EXAFS data from Am-Aquo , we initially calculated (FEFF8 (ref. 32 )) an EXAFS spectrum using atomic coordinates obtained from the [Am(H 2 O) 9 ][O 3 SCF 3 ] 3 single-crystal X-ray diffraction data, previously reported [33] . The calculated EXAFS spectrum was composed of two main scattering pathways. The first path originated from six oxygen atoms with an Am − O H 2 O distance of 2.465 Å and the second path had three oxygen atoms at 2.578 Å. Although various EXAFS fitting parameters were considered based on these calculations, only one oxygen shell could be resolved in the experimental data, as our resolution between k of 2.6 and 12 was only 0.167 Å ( π /2Δ k ). The final model of the EXAFS data with the lowest residual factor and reduced chi-squared value consisted of 9.5±0.9 oxygen atoms at 2.48(1) Å ( Table 1 and Figs 2 and 3 ). These Am − O H 2 O bond distances and CNs were consistent with the Am(H 2 O) 9 3+ solid-state structure and EXAFS spectra previously obtained on Am III aquo ions in different solvent matrices, for example, Stumpf et al . [34] in 0.025 M HClO 4 and Allen et al . [35] in 0.25 M HCl ( Table 1 ). Table 1 Structural parameters determined using solution-phase EXAFS. 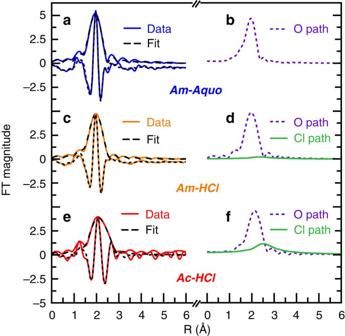Figure 3: Fourier Transform of the AcIIIand AmIIIk3-EXAFS. (a) Fourier Transform ofk3-EXAFS spectra fromAm-Aquo(0.11 M HO3SCF3) in blue trace and its fit in dashed black trace. (b) Oxygen path contribution in the fitted data in dashed purple. (c) Fourier Transform ofk3-EXAFS spectra fromAm-HCl(11 M HCl) in red trace and its fit in dashed black trace. (d) Oxygen and chlorine paths contribution in the fitted data in dashed purple and green solid trace, respectively. (e) Fourier Transform ofk3-EXAFS spectra fromAc-HCl(11 M HCl) in red trace and its fit in dashed black trace. (f) Oxygen and chlorine paths contribution in the fitted data in dashed purple and green solid trace, respectively. Full size table Figure 3: Fourier Transform of the Ac III and Am III k 3 -EXAFS. ( a ) Fourier Transform of k 3 -EXAFS spectra from Am-Aquo (0.11 M HO 3 SCF 3 ) in blue trace and its fit in dashed black trace. ( b ) Oxygen path contribution in the fitted data in dashed purple. ( c ) Fourier Transform of k 3 -EXAFS spectra from Am-HCl (11 M HCl) in red trace and its fit in dashed black trace. ( d ) Oxygen and chlorine paths contribution in the fitted data in dashed purple and green solid trace, respectively. ( e ) Fourier Transform of k 3 -EXAFS spectra from Ac-HCl (11 M HCl) in red trace and its fit in dashed black trace. ( f ) Oxygen and chlorine paths contribution in the fitted data in dashed purple and green solid trace, respectively. Full size image The EXAFS fitting results can be interpreted using static or dynamic descriptions. A static interpretation suggested that the americium aquo ion had 9.5 H 2 O ligands held at a fixed 2.48(1) Å distance. In contrast, the dynamic interpretation described the EXAFS data as an averaged spectrum from a heterogeneous mixture over the lifetime of the experiment. In this scenario, the number of H 2 O molecules in the Am III inner coordination sphere varied, as did the Am − O H 2 O distances. To provide insight, MD-DFT calculations were carried out on a single Am III ion inside a box (12.54 × 12.45 × 12.68 Å 3 ) of explicit H 2 O (64 total) solvent molecules. Before the simulation, the components of the box were randomized (see Methods), and then the MD were modelled for 330 fs. The MD trajectory showed a time average of 8.1±0.3 H 2 O molecules within a 4 Å radius of the Am III ion. The average Am − O H 2 O distances were displayed by the red solid traces in Fig. 4 . At the start of the calculations the variation in Am − O H 2 O bond distances were large, ranging from 2.7 to 2.5 Å. However, after ∼ 50 fs, the magnitude of these oscillations became smaller and centred ∼ 2.5 Å. In general, these calculations were in excellent agreement with the EXAFS experiment. Both theory and experiment identified a CN around nine and the calculated average Am − O H 2 O distances bracketed the experimental value (red dashed trace). The good agreement of the Am-Aquo experimental and computational EXAFS analyses with the single-crystal and solution-phase EXAFS studies provided confidence and credibility that our methods could be applied accurately to other actinide systems. 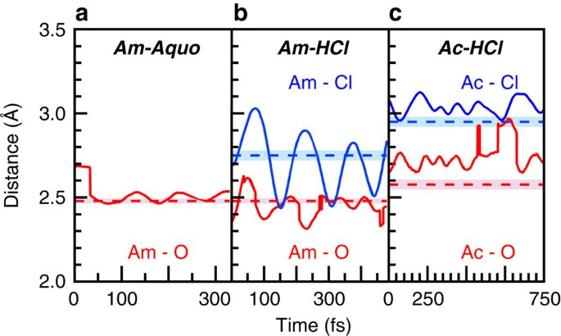Figure 4: MDDFT calculations. The calculated meanM-OH2O(solid red traces) and M–Cl (solid blue traces) distances for O and Cl atoms within 4 Å of the metal (Am or Ac) have been compared with the values obtained from the experimental EXAFS analyses (M-OH2Odashed red and M–Cl dashed blue traces with their associated errors bars represented as shaded boxes). Experimental errors bars were 0.01 or 0.03 Å. SeeTable 1. (a) Data forAm-Aquo, (b) Data forAm-HCland (c) Data forAc-HCl. Figure 4: MDDFT calculations. The calculated mean M-O H 2 O (solid red traces) and M–Cl (solid blue traces) distances for O and Cl atoms within 4 Å of the metal (Am or Ac) have been compared with the values obtained from the experimental EXAFS analyses ( M-O H 2 O dashed red and M–Cl dashed blue traces with their associated errors bars represented as shaded boxes). Experimental errors bars were 0.01 or 0.03 Å. See Table 1 . ( a ) Data for Am-Aquo , ( b ) Data for Am-HCl and ( c ) Data for Ac-HCl . Full size image To obtain atomic coordinates for modelling the Am-HCl data, we calculated EXAFS spectra using FEFF8 from two different sources. The first model employed atomic coordinates from previously reported [AmCl 2 (H 2 O) 6 ]Cl single-crystal X-ray diffraction data [36] , which had two Cl 1– and six H 2 O inner-sphere ligands. The second simulation utilized a DFT-optimized structure of AmCl 2 (H 2 O) 4 1+ . Refinement of the experimental EXAFS data using fitting parameters from either model converged to the same point ( Table 1 and Figs 2 and 3 ), showing an approximate nine-coordinate Am III ion with 0.8±0.3 Cl 1– and 8.3±0.9 H 2 O molecules in the inner sphere. Although the contributions from Cl 1– to the overall EXAFS spectrum seemed slight ( Fig. 3 ), omitting the Cl 1– shell provided a significantly worse model, by over 91% confidence as determined from the Hamilton statistical test [37] . The measured americium coordination environment seemed reasonable when compared with other solution-phase EXAFS studies. For instance, our Am-HCl CNs—collected in HCl solutions of 11 M—were bracketed by those determined from solutions with lower and higher Cl 1– concentrations ( Table 1 ). Allen et al .’s EXAFS experiments at lower HCl solutions (0.25 M) showed no inner-sphere Cl 1– ligands, while those at higher Cl 1– concentrations—a mixture of HCl (0.25 M) and LiCl (12.5 M)—showed 1.8 Cl 1– ligands [35] . When experimental errors were considered, our data also agreed with measurements conducted at similar Cl 1– concentrations, for example, Allen et al . identified 1.2 Cl 1– ligands in solutions containing mixtures of HCl (0.25 M) and LiCl (10.0 M) (ref. 35 ). Our 2.75(3) Am–Cl and 2.48(1) Am − O H 2 O distances also agreed with metrics from the solid-state single-crystal X-ray diffraction study, 2.799(2) and 2.462(9) Å, respectively [36] , and were consistent with Allen et al .’s solution-phase EXAFS results in LiCl (10.0 M, 12.5 M); which had Am–Cl distances between 2.80 and 2.81 Å and Am − O H 2 O distances varying from 2.48 to 2.51 Å [35] . These Am-HCl EXAFS results agreed with the MD-DFT calculations. The calculations were conducted similarly to those described above for Am-Aquo , with the exception that one Cl 1– anion was included in the calculation. Over the course of 480 fs, we calculated an average of 1 Cl 1– and 8.05±0.9 H 2 O molecules within a radius of 4 Å from the Am III ion. The average Am–Cl and Am − O H 2 O distances were quite similar to the experimental EXAFS values as shown in Fig. 4 . Given the paucity of actinium structural studies [38] , [39] , the DFT and MD-DFT calculations proved useful in guiding the interpretation of the EXAFS spectrum from Ac-HCl . Atomic coordinates for the EXAFS refinement were obtained from MD-DFT calculations on AcCl 3 (H 2 O) 5 . The resulting EXAFS analysis identified two unique scattering paths; one associated with the H 2 O ligands composed of 6.6±1.8 molecules at 2.59(3) Å and a second at 2.95(3) Å consisting of 3.2±1.1 Cl 1– ligands (Debye–Waller factor=0.0074 Å 2 ; Figs 2 and 3 ). These bond distances were in excellent agreement with the sum of the Ac III and Cl 1- ionic radii, 1.12 Å+1.81 Å=2.93 Å (ref. 40 ). If the chlorine path was ignored and only the oxygen path used, the quality of the fit decreased (>93% confidence based on the Hamilton’s statistical test [37] ), gave a high Debye–Waller factor value (0.018 Å 2 ), and provided an unrealistic number of coordinated H 2 O molecules (14 total). The Ac-HCl experimental data agreed well with MD-DFT calculations conducted on a box containing one Ac III , three Cl 1– ligands and 64 H 2 O molecules for 1 ps. The MD-DFT revealed all three Cl 1- and 6.14±0.34 H 2 O ligands within 4 Å of the Ac III ion for the duration of the calculation. The average Ac − O H 2 O and Ac–Cl distances were calculated to be 2.76±0.08 and 3.04±0.13 Å, respectively. Although the magnitudes of these values were larger than that determined experimentally (by 0.17 Å for Ac − O H 2 O and 0.09 Å for Ac–Cl), the calculated and experimental results agreed within 1 σ for the Ac–Cl, and 2 σ for the Ac − O H 2 O . Such deviations between theory and experiment were not unusual and have been observed in calculations on other systems that employed the generalized gradient approximation functional. The calculated CNs also agreed with the experimental values, showing ∼ 3 Cl 1– and ∼ 6 H 2 O inner-sphere ligands. We note that the agreement between experiment and theory was better in the two americium cases described above. It was possible that these subtle differences between theory and experiment resulted from the low signal-to-noise at high k in the experimental Ac L 3 -edge EXAFS spectrum, as the actinium concentrations were appreciably smaller than americium (μM versus mM). Alternatively, it was possible that the behaviour of Ac III was more difficult to model, as the fundamentals of actinium have been less well defined than those of americium. Regardless, both theory and experiment indicated substantial differences between the Ac III and Am III coordination environments in HCl solutions, which represented an unexpected variation in actinide(III) reactivity. It is this observation that has inspired our future efforts to better understand the origin for diverging Ac III versus Am III -binding preferences. The experimental and computational results described here represented an exciting leap forward from previous actinium coordination chemistry studies. To most effectively communicate to the reader the significance of these results, we found it instructive to summarize the previous Ac III coordination chemistry. The majority of actinium chemistry has been inferred from methodical radio-analytical and extraction studies conducted on trace-level quantities of actinium [39] , [41] , [42] , [43] . Although these previous efforts revealed differences between Ac III and the other trivalent actinide and lanthanide elements, in general, they have been interpreted as suggesting that Ac III is a hard oxophilic tri-cation, in direct analogy to other actinide(III) cations. In addition, there have been a few studies that used macroscopic quantities of Ac III for analysis by ultraviolet–visible spectroscopy [43] , [44] . However, these spectra were essentially featureless—owing to the actinium 5 f 0 6 d 0 ground-state electronic configuration—and did not provide an insight into the actinium coordination environment. The majority of actinium structural data was obtained during the Manhattan project and through the years shortly after World War II. For example, Fried et al . [38] and Zachariasen [45] , [46] , [47] deduced structures and cell parameters using X-ray diffraction patterns from crystalline powders of nine actinium compounds assumed to be AcF 3 , AcCl 3 , AcBr 3 , Ac 2 O 3 , Ac 2 S 3 , AcOF, AcOCl, AcOBr and AcPO 4 ·H 2 O. Subsequently, Farr et al . used X-ray diffraction to characterize microgram quantities of a mixture of actinium metal and actinium hydride [48] . Years later, an attempt to prepare some inorganic compounds with 10 mg of 227 Ac occurred. Unfortunately, radiation damage to samples and the diffraction films limited this effort to generate a single powder pattern of actinium oxalate, Ac 2 (C 2 O 4 ) 3 ·10H 2 O (ref. 49 ). Reported here, we overcame some of the challenges associated with spectroscopic analyses of bulk actinium samples using new XAFS capabilities, which have been typically employed in trace-level environmental science studies. Briefly, we characterized the chemistry of Ac III and Am III in concentrated HCl (11 M) solutions and compared the results with solution-phase measurements from the americium aquo ion in dilute HO 3 SCF 3 (0.11 M). Calculations involving MD-DFT, previously reported single-crystal X-ray diffraction, and previous solution-phase EXAFS results (when possible) were employed to guide our spectral interpretations. These efforts enabled the Ac–Cl and Ac − O H 2 O distances to be directly measured for the first time. Moreover, the studies revealed a substantial difference between Ac III and Am III solution speciation. In concentrated HCl solutions, we observed that Ac III and Am III were coordinated by approximately nine ligands; however, Ac III preferred approximately six H 2 O molecules and three Cl 1– ions, while Am III was coordinated by approximately eight H 2 O and one Cl 1– ligands. It is well known that evaluating CN using EXAFS typically provides values with high uncertainty, ∼ 20%. In spite of the large errors associated with the Ac III (CN Cl =3.2±1.1) and Am III (CN Cl =0.8±0.3) chloride CNs, these values clearly indicated that Ac III had more Cl 1- ligands in the inner coordination sphere than Am III . These results were indeed unexpected, for example, stability constants for Ac–Cl and Am–Cl were reported to be nearly identical [6] . Perhaps differences in steric crowding accounted for the varied H 2 O and Cl 1– CNs for the large Ac III versus smaller Am III ions ( Fig. 5 ). However, Ac III electronic structure contributions may also contribute to difference in H 2 O versus Cl 1– binding. While the generality and origin of these results have yet to be established, they tempt us to revisit the traditional descriptions of Ac III . For example, consider the possibility that Ac III is substantially less polarizing than the rest of the f -elements, which are well established as hard and oxophilic ions. In this sense, one might crudely compare the changes in chemical hardness from Ac III to Am III to that of iodine to fluorine. It is conceivable that a reclassification could provide insight into previous reports where actinium behaved substantially different than trivalent actinides and lanthanides [41] , [42] . Given that many Ac III chelators are based on the coordination chemistry of lanthanides and minor actinides, better characterization of the long Ac–ligand bond distances, binding preferences, and speciation has the potential to improve design parameters for actinium chelators. In this context, the results here serve as motivation for future work focused on using XAFS spectroscopy and MD-DFT calculations to advance understanding of actinium reactivity with ligands that are more relevant to α-therapy development. 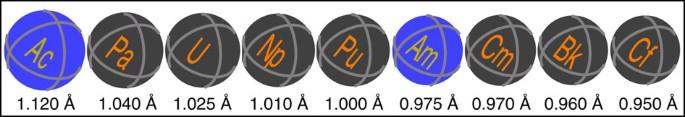Figure 5: Ionic radii of the early to mid-actinides. Scheme showing the ionic radii (Å) of trivalent actinides from actinium to californium drawn to scale for six-coordinate ions40. Figure 5: Ionic radii of the early to mid-actinides. Scheme showing the ionic radii (Å) of trivalent actinides from actinium to californium drawn to scale for six-coordinate ions [40] . Full size image General consideration Caution! The 243 Am and 227 Ac isotopes α-, β- and γ-emitting radionuclides have high specific activity and decay to α-, β- and γ-emitting isotopes. Hence, this research was conducted in a radiological facility with appropriate analyses of these hazards and implementation of controls for the safe handling and manipulation of these toxic and radioactive materials. All direct handling of these radionuclides was conducted within certified fume hoods and monitored with appropriate α-, β- and γ-particle detecting instruments. The 227 Ac and 243 Am isotopes were supplied by the United States Department of Energy Office of Science Isotope Program in the Office of Nuclear Physics. Hydrochloric acid and trifluoromethanesulfonic acid were obtained commercially (Fisher Scientific). Water was purified to 18.2 MΩ/cm resistivity using Thermo-Scientific Barnstead Nanopure or Millipore Nanopure water purification systems. Resins used for separations—DOWEX AG1-X8 (BioRad; 100–200; Cl form) and branched DGA (Eichrom)– were suspended in water, and the fines decanted before use. Separations were characterized using γ-spectroscopy using an EG&G Ortec Model GMX-35200-S HPGe detector system in combination with a Canberra Model 35-Plus multichannel analyser associated with Gamma Vision software. Characterization was also performed using α-spectroscopy with and Ortec Octete+ α-spectrometer associated with Ortec Alpha Vision analytical software to control the spectrometer, to acquire and analyse the data. Sample preparation The coordination chemistry studies described herein made use of 227 Ac (2 mCi; 28 μg) and 243 Am (0.5 mg per sample). Safety concerns regarding the radiation dose from the 227 Ac sample were mitigated by removing the 227 Ac daughters (primarily 227 Th and 223 Ra) the day before shipping to the SSRL synchrotron facility and by completing the measurements before significant quantities of the 227 Ac daughters re-emerged, ∼ 10 days from separation. Given the scarcity of 227 Ac and 243 Am, these actinide isotopes were recycled after the XAFS data collections. In the case of actinium, the sample matrix was converted from HCl to HNO 3 (8 M) and the actinium was recovered and purified using the chromatographic procedures described below [26] , [27] . For americium, samples were recovered and purified using cation exchange chromatography [50] . In general, the samples were dissolved in dilute acid (five drops HCl in 5 mL H 2 O) and loaded onto a Biorad column (10 ml) charged with AG50x8 resin (2 ml) that had been conditioned with HCl (1 M; 5 × 10 ml). The column was washed with HCl (0.1 M; 6 × 10 ml), and americium was eluted from the column using concentrated HCl (12 M; 5 × 5 ml). The recovered actinium and americium samples were analysed by γ-spectroscopy to confirm isotopic purities and the americium samples by ICP-AES to confirm chemical purities. Actinium-227 samples Using previously established methods [26] , [27] , radiochemical purification of 227 Ac was accomplished by exploiting oxidation state differences between the Ac III parent and the tetravalent (Th IV ) and divalent (Ra II ) daughters ( Fig. 6 ). The 227 Ac isotope, and its daughters, were dissolved in HNO 3 (1 ml; 8 M). The solution was loaded using HNO 3 (4 × 1 ml; 8 M) onto a Biorad column charged with an anionic exchange resin (1 ml, AG1-X8, BioRad). The resin had been conditioned with H 2 O (5 × 3 ml), HNO 3 (5 × 3 ml 8 M), H 2 O (1 × 2 ml) and HNO 3 (3 × 3 ml 8 M). Under these conditions, 227 Ac, 223 Ra, 211 Pb and 211 Bi, eluted from the column during the load and with subsequent washes with HNO 3 (10 ml; 8 M). Meanwhile 227 Th was retained on the resin. The eluted 227 Ac fractions were combined and diluted with water by a factor of two, such that the resulting solution contained HNO 3 (4 M). The solution was loaded onto a Biorad column charged with branched DGA resin (1 ml). The resin has been conditioned with HNO 3 (3 × 2 ml; 0.05 M) followed by HNO 3 (3 ml; 4 M). Under these conditions, 223 Ra eluted while 227 Ac remained bound to the resin. The resin was washed with HNO 3 (3 × 2 ml; 4 M). Subsequently, 227 Ac was eluted using with HNO 3 (4 × 2 ml; 0.05 M). The 227 Ac concentration was determined by γ-spectroscopy to be highest in the first two fractions. The 227 Ac fractions were combined and the solution evaporated in a conic shape glass vial on a hot plate under a slow stream of air to a soft dryness. The solid residue was converted from NO 3 1− to Cl 1− to generate a solution of actinium in concentrated HCl by repeated evaporation and dissolution in HCl (11 M; 2 × 2 ml). The solid residue was then dissolved in HCl (0.455 ml; 11 M) and transferred to the XAFS holder. 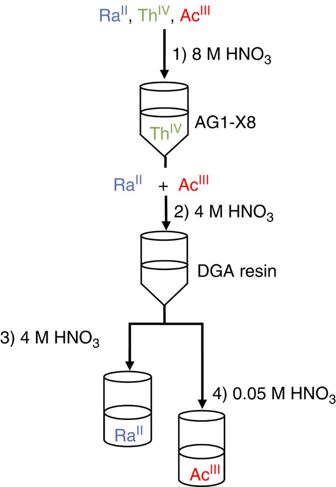Figure 6: Cartoon describing227Ac radiochemical purification. Scheme showing the procedure followed to separate227Ac from its daughters229Th and223Ra using anion exchange resin and DGA resin, respectively. Figure 6: Cartoon describing 227 Ac radiochemical purification. Scheme showing the procedure followed to separate 227 Ac from its daughters 229 Th and 223 Ra using anion exchange resin and DGA resin, respectively. Full size image Americium-243 samples Americium samples in either HCl (11 M) or HO 3 SCF 3 (0.11 M) acidic solutions were prepared from a stock of AmO 2 dissolved in HCl (6 M). Solutions of americium in HCl (11 M) were generated in direct analogy to the method described above for actinium. Briefly, an aliquot from an 243 Am stock solution containing Am III (0.6875, mg) in HCl (0.250 ml; 6 M) was heated to dryness in a glass vial in a sand bath on a hot plate. The solid was then dissolved in concentrated HCl (0.5 ml; 11 M) and this evaporation/dissolution process was repeated two more times. The resulting solid residue was dissolved (peach colour) in HCl (0.455 ml; 11 M) and transferred to the XAFS holder. The solution containing americium aquo ion was prepared from an aliquot of an 243 Am stock solution containing Am III (0.6875, mg) dissolved in HCl (0.250 ml; 6 M). The solvent was removed by heating the solution in a glass vial in a sand bath on a hot plate. The solid residue was then dissolved in Millipore H 2 O and transferred to an Eppendorf tube (2 ml volume). Quickly, NaOH (0.050 ml; 2 M) was added, the solution shaken, and centrifuged for 3 min (6,000 r.p.m.). The supernate was decanted from the resulting pink precipitate and discarded. The solid was washed with NaOH (2 × 0.06 ml; 10 mM) and with Millipore H 2 O. The solid precipitate was then dissolved in trifluoromethanesulfonic acid (0.455 ml; 0.11 M) and transferred to the XAFS holder. XAFS Sample preparation All XAFS samples were loaded into XAFS cells that were triply contained, which protected against release of radiological material during samples shipment and XAFS experiments. The XAFS holder consisted of a plastic holder body with a 2 mm well equipped with a set of Teflon and a Kapton windows (1 mil). Solutions were introduced into the holder through an injection hole sealed with a gasket that was held in place by an aluminium plate. The sample cell holder was then transferred into the secondary and the tertiary container, which were best described as a set of nested aluminium holders equipped with Kapton windows (2 mil). XAFS measurements The XANES and EXAFS were measured at SSRL under dedicated operating conditions (3.0 GeV, 5%, 500 mA) on end station 11-2. This beamline was equipped with a 26-pole, 2 Tesla wiggler, utilized a liquid nitrogen-cooled double-crystal Si[220] monochromator and employed a collimating and focusing mirrors. A single energy was selected from the white beam with a liquid-N 2 -cooled double-crystal monochromator utilizing Si[220] ( ϕ =0) crystals. The crystals were run de-tuned by 35%, ∼ 500 eV above the absorption edge to eliminate higher harmonics from the monochromatic light. The samples were attached to the beamline 11-2 XAFS rail. The rail was equipped with three ionization chambers through which nitrogen gas was continually flowed. One chamber was positioned before the sample holder, to monitor the incident radiation ( I 0 , 10 cm). The second chamber was positioned after the sample holder, such that sample transmission ( I 1 , 30 cm) could be evaluated against I 0 , while a third chamber ( I 2 , 30 cm) positioned downstream from I 1 , so that the XANES of a calibration foil could be measured in situ during the XAFS experiments against I 1 . Conditions for the americium aqua ion sample was also optimized for transmission data collection. Actinium and americium solution samples in concentrated HCl were measured in fluorescence mode using solid-state 100-Ge element detector against the incident radiation ( I 0 ). Low-energy contributions to the fluorescence signal were removed using a bromine filter (three path lengths) for actinium and yttrium (three path lengths) for americium. Before measurements, dead-time correction measurements were performed at ∼ 400 eV above the element edge of the filter. The dead time correction curve corresponds to the plot of the windowed counts of the emission line of interest versus the total of incoming counts in the solid-state detector. This procedure was performed by putting filters (Se for Ac and Sr for Am) in front of the fluorescence detector. XAFS data analysis Data manipulation and analysis was conducted as previously described [51] . First the data were dead-time corrected and calibrated to the energy of the first inflection point of the calibration foil measured in situ . The measurements were calibrated as follows. For actinium, a RbCl pellet was prepared by sandwiching RbCl diluted with BN to a one absorption length thickness. The energy for the first inflection point was determined in comparison with the Bi L II -edge (15,711 eV) to be 15,203.81 eV. Americium samples were calibrated to a zirconium foil at 17,998 eV. Data from the analytes were analysed by fitting a line to the pre-edge region, which remove the background from experimental data in the spectra. Then a second- to third-order polynomial fitting was chosen for the post-edge region. The difference between pre- and post-edge lines is set to unity at the first inflection point, normalizing the absorption jump to 1.0. Each of the samples were measured for several hours resulting in the collection of 25 scans for Ac and five scans for Am. Fittings using ATHENA and ARTEMIS [52] were performed using crystallographic data from americium triflate [33] , americium trichloride hexahydrate [36] and FEFF8 calculations [32] . The spectra were fitted using only single-scattering paths obtained from FEFF8. The adjustments of spectra were performed in different k and R ranges for each samples, where R is the distance to the neighbouring atom; americium triflate was adjusted in 2.6< k <12 Å –1 and 1.25< R <3 Å, americium in concentrated HCl in 2.6< k <10.5 Å –1 and 1.1< R <3.5 Å and actinium in concentrated HCl in 2.6< k <9 Å –1 and 1.2< R <3.45 Å. For the fitting procedure, the CN, the distance ( R ) and the Debye–Waller factor ( σ 2 ) were allowed to vary but for the last factor a single value was chosen for both paths used for the first shell. A single value of energy shift (Δ E 0 ) was used for all scattering paths. The amplitude reduction factor (S 0 2 ) was set at 0.9 based on initial fits. MD-DFT calculations The Born–Oppenheimer MD simulations in the Helmholtz ensemble (NVT) were performed using the computer code VASP (Vienna Ab-initio Simulations Package) [53] version 5.35. In this code, the forces on the ions are calculated from the electronic structure of the whole system computed using DFT at the generalized gradient approximation level using the functional by Purdue–Burke–Enzerhof [54] . A simulation box of (12.54 × 12.45 × 12.68 Å 3 ) was used, including the metal ion (M 3+ ), three Cl 1− counter-ions maintained the simulation box neutral, and for solvent medium we used 64 water molecules. However, for the simulations of the single aquo ion no counter-ions were added to the system and a uniform background charge of −3 was added to keep the neutrality of the simulation box. The basis set consists in an expansion into plane-wave functions. Because of the large size of the simulation box, the k -space representation included only the Γ point. The energy cutoff for the plane-wave expansion was set at 500 eV and scalar relativistic effects were included using the PAW-PBE potentials [55] . Initially the metal ion and the closest neighbouring molecules and counter ions were kept frozen and the solvent plus remaining counter-ion atoms were heated up to 498 K to be thermalized for 1 ps. After that a 1 ps run was done at 298 K with all the degrees of freedom released to thermalize the complex with the solvent. Finally a 1 ps data collection run was performed where we monitored the solvent and ion dynamics. Data availability The data that support the findings of this study are available within the article or from the corresponding authors on request. How to cite this article: Ferrier, M. et al . Spectroscopic and computational investigation of actinium coordination chemistry. Nat. Commun. 7:12312 doi: 10.1038/ncomms12312 (2016).